Optical measurements of long-range protein vibrations Protein biological function depends on structural flexibility and change. From cellular communication through membrane ion channels to oxygen uptake and delivery by haemoglobin, structural changes are critical. It has been suggested that vibrations that extend through the protein play a crucial role in controlling these structural changes. While nature may utilize such long-range vibrations for optimization of biological processes, bench-top characterization of these extended structural motions for engineered biochemistry has been elusive. Here we show the first optical observation of long-range protein vibrational modes. This is achieved by orientation-sensitive terahertz near-field microscopy measurements of chicken egg white lysozyme single crystals. Underdamped modes are found to exist for frequencies >10 cm −1 . The existence of these persisting motions indicates that damping and intermode coupling are weaker than previously assumed. The methodology developed permits protein engineering based on dynamical network optimization. Well-known biological processes rely on protein structural changes, such as neuron signal transmission and oxygen transport. The opening and closing of ion channels for signalling currents depends on the structural changes of the transmembrane protein forming the pore [1] . In the case of haemoglobin, the oxygen-transporting protein in blood, global structural change with initial binding of oxygen in a single domain biases the structure towards binding in additional domains, increasing delivery efficiency [2] . It has long been speculated that protein structural change critical to function is mediated through long-range vibrational motions involving dynamical networks extending throughout the protein [3] , [4] , [5] . Drastic changes in enzyme efficiency [6] , [7] , [8] , and electron transfer rates [9] with mutations remote from the active site have been attributed to these long-range motions linking the mutation site with the active site. The relevance of protein intramolecular motions to function was first inferred from calculations showing that functional conformational change is replicated using only the first few lowest energy vibrational modes for a variety of systems [10] , [11] , and reports of reaction rate control by optical overpumping [12] . Inelastic scattering measurements have indicated these motions are present [13] , [14] but the measurements required complex facility-based methods as well as cryogenic temperatures and/or non-physiological hydrations. The lack of measurement of these motions under physiological conditions has led to the assumption that the similarity between the calculated motions and protein functional structural change merely indicates a dynamic predisposition towards the functional intermediate states and that the motions themselves do not exist but are overdamped. The measurement of protein long-range vibrations are challenged in part by the dense nearly featureless vibrational density of states (VDOS), which is peaked in the terahertz frequency range (0.03–6.0 THz, 1–200 cm −1 , 12.5 μeV–25 meV) [15] , [16] , [17] . Optical measurements can reduce this complexity by selecting modes that have a strong interaction with light: that is strong dipole coupling. However, standard THz spectroscopic techniques have been unsuccessful in isolating specific modes because of a large additional glass-like background from librational motions of the solvent and peptide side chains [18] , [19] , [20] , [21] , [22] , [23] . Here we achieve high mode contrast by utilizing the property that the glass-like background is isotropic, whereas the dipole coupling to protein collective modes will be dependent on the protein orientation relative to the light polarization. Taking the difference in the measured absorbance for different light polarizations removes the isotropic background and enhances the contrast between the anisotropic collective mode absorbances. This approach requires samples where the molecules are in an ordered array, for example, protein crystals. However, protein crystals are typically much smaller than the diffraction limited spot size at THz frequencies. We overcome the limitation by using a near-field THz microscopy method we refer to as crystal anisotropy terahertz microscopy (CATM). We find strong orientation and hydration-dependent resonances for chicken egg white lysozyme (CEWL) tetragonal crystals. Further, initial calculations suggest that the two lowest energy resonant features observed involve structural motion at the binding site. 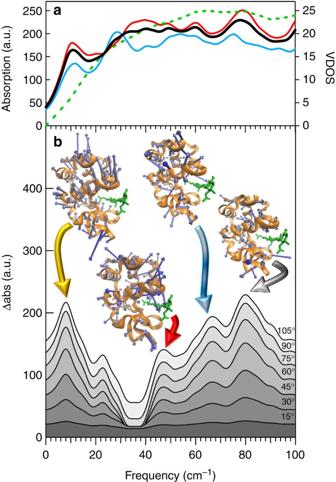Figure 1: Calculations of the structural vibrations for hydrated CEWL. (a) Specific mode identification is not possible from the dense smooth VDOS (dashed green line). The dipole coupling necessary for optical absorbance reduces the number of modes that contribute to the absorption, thereby allowing for sharper frequency-dependent features, shown in black for unaligned molecules. Contrast increases further for optical absorbance of aligned molecules and polarized light. This is shown for a tetragonal crystal of CEWL. The blue curve indicates the calculated absorption for the electric field polarization parallel to the (001) crystal axis. The red curve indicates the calculated absorption for the electric field polarization parallel to the (−110) crystal axis. However. a strong isotropic glass-like contribution, not shown, obscures this structure for measurements at a single polarization. The background can be removed by subtracting the absorbance for different polarization directions. (b) The calculated Δabs for different protein crystal orientations. Each curve is offset by 20 units for clarity. By measuring Δabs, the isotropic background is removed and structural mode identification is possible. Specific correlated protein motions corresponding to several of the Δabs peaks are represented by the molecular diagrams. The displacement vectors (blue, calculated using NMA) indicate concerted motion throughout the macromolecule (yellow) for these vibrational modes. In particular, the motions associated with the peaks at 8 and 47 cm−1involve expansion and compression at the substrate-binding site, indicated by the inhibitor (green). Normal mode analysis Figure 1a shows the calculated VDOS for a single CEWL molecule with 92 waters included. The VDOS (dashed green line) is smooth over this frequency range showing that identification of specific structural modes is not possible from the VDOS. Also shown is the calculated THz light absorbance for an unaligned sample (black solid line) where the absorbance is averaged over all polarization directions. While still smooth, the unaligned absorption has distinct features at 11 and 80 cm −1 reflecting the absorbance sensitivity to the dipole-coupling strength of the modes. In typical THz measurements of CEWL powder, hydrated films, solutions and crystals these distinct modes have not been observed [24] , [25] , [26] , [27] . This is likely due to the dominance of the librational and relaxational response of the water and side chains not included in the calculation in Fig. 1a . Also presented is the calculated absorbance for a tetragonal CEWL crystal with negligible crystal contact forces for light incident on the (110) face. The absorbance is shown for the polarization parallel to the [001] and [−110] crystal directions. There is a clear difference in the spectra for the two polarization directions. The glass-like background, not included in these calculations, would be the same for both polarizations; thus, by taking the difference in the measured absorbance, this background is removed. That is, the absorption for a polarization direction is abs( )=abs anisotropic ( )+abs isotropic , so the isotropic background is removed by measuring the absorption for different polarization directions and determining the change in absorption relative to a single reference direction: Δabs=abs( )− abs( ref ). For the measurements discussed here, the THz light is incident on the (110) crystal face, with the terahertz polarization vector lying in the plane perpendicular to [110]. Figure 1b shows the calculated Δabs=abs( )− abs([001]), as the polarization direction rotates from the [001] direction to the [−110] direction. Several peaks strengthen with rotation, corresponding to the increase in absorption for these modes. As will be shown, the peaks at 8, 23, 47, 69 and 80 cm −1 correlate well with measurements. The displacement vector diagrams for modes associated with four of these peaks are shown on the diagram. The displacements show correlated motion throughout the macromolecule at these frequencies. Of particular interest is how these global motions affect activity. In the case of CEWL, its function is to attack cell walls by cleaving carbohydrates within the membrane. In Fig. 1b , the CEWL inhibitor tri- N -acetylglucosamine (green) illustrates the carbohydrate-binding site (also known as the substrate-binding site) in the protein. One can see that the correlated motion indicated by the displacement vectors for the 8 and 47 cm −1 peak modes directly affects access to the binding site and the clamping down on the substrate associated with the enhanced interaction for cleaving of the bonds. Figure 1: Calculations of the structural vibrations for hydrated CEWL. ( a ) Specific mode identification is not possible from the dense smooth VDOS (dashed green line). The dipole coupling necessary for optical absorbance reduces the number of modes that contribute to the absorption, thereby allowing for sharper frequency-dependent features, shown in black for unaligned molecules. Contrast increases further for optical absorbance of aligned molecules and polarized light. This is shown for a tetragonal crystal of CEWL. The blue curve indicates the calculated absorption for the electric field polarization parallel to the (001) crystal axis. The red curve indicates the calculated absorption for the electric field polarization parallel to the (−110) crystal axis. However. a strong isotropic glass-like contribution, not shown, obscures this structure for measurements at a single polarization. The background can be removed by subtracting the absorbance for different polarization directions. ( b ) The calculated Δabs for different protein crystal orientations. Each curve is offset by 20 units for clarity. By measuring Δabs, the isotropic background is removed and structural mode identification is possible. Specific correlated protein motions corresponding to several of the Δabs peaks are represented by the molecular diagrams. The displacement vectors (blue, calculated using NMA) indicate concerted motion throughout the macromolecule (yellow) for these vibrational modes. In particular, the motions associated with the peaks at 8 and 47 cm −1 involve expansion and compression at the substrate-binding site, indicated by the inhibitor (green). 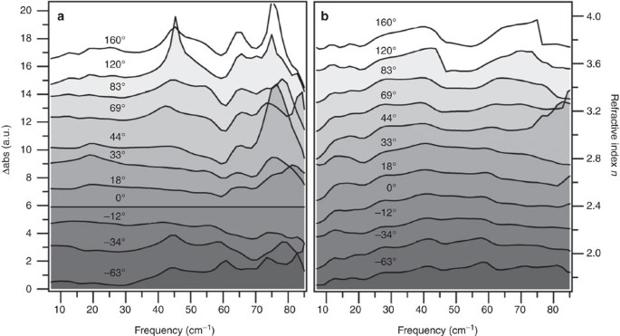Figure 2: CATM measurements of a dry CEWL crystal. (a) Δabs measurements show strong narrow resonances that grow in and diminish as the crystal is rotated. (b) The measured index has anomalous dispersion at the same frequencies as Δabs peaks, consistent with resonant absorption. Full size image Dehydrated CEWL collective mode measurements Figure 2a shows our Δabs measurements for a dry CEWL tetragonal crystal. Relative orientations of the protein crystal are determined by an indicator on the sample plate; however, the imaging system used for these measurements did not have sufficient magnification to determine the absolute crystal axis orientation relative to the THz polarization. This limitation is readily overcome with additional instrumental development. The zero-angle reference measurement was chosen arbitrarily. There are several clear orientation-dependent resonances at 19, 45 and 60 cm −1 . In Fig. 2b , we show the refractive index from the same measurements, using the transmission through the empty aperture as an absolute reference for index determination. The classic anomalous dispersion occurring at the same frequencies as the strong absorbance features in Fig. 2a confirms that the features are indeed absorbance resonances. This is the first time that sharp absorbance lines have been measured for a protein sample at THz frequencies that clearly arise from the sample and not from multiple reflection artifacts. Figure 2: CATM measurements of a dry CEWL crystal. ( a ) Δabs measurements show strong narrow resonances that grow in and diminish as the crystal is rotated. ( b ) The measured index has anomalous dispersion at the same frequencies as Δabs peaks, consistent with resonant absorption. Full size image Hydrated CEWL collective mode measurements A surface plot of the hydrated CEWL crystal CATM measurements are shown in Fig. 3a . The 45 cm −1 resonance seen in the dry crystal is still present for the hydrated crystal; however, the 19 and 60 cm −1 resonances are no longer present. New resonances are observed at 12, 20, 69 and 78 cm −1 for the hydrated crystal. The resonance linewidths for the hydrated crystal are narrower than the dehydrated crystal. A comparison of the linewidths between the dehydrated and hydrated crystals is shown in the Supplementary Fig. 1 . There are several possible origins of this broadening for the dehydrated crystal. First, the relative alignment of the proteins slightly decreases with dehydration and second, the protein conformation may not be uniform throughout the dehydrated crystal owing to varying water content. The expected change in crystal packing is slight, but may be sufficient to result in this broadening [28] . 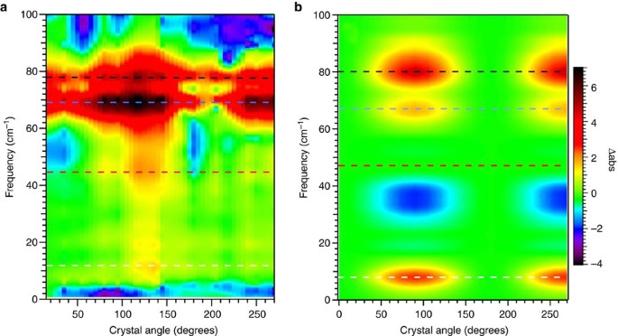Figure 3: Surface plots of Δabs versus protein crystal orientation angle and frequency. (a) Hydrated CEWL crystal CATM measurements. (b) Hydrated CEWL crystal normal mode calculations. The measurements show the same periodicity as predicted by the calculations. The dashed lines indicate frequencies where measured periodic peaks have frequencies similar to periodic peaks in the calculations. The calculated 47 cm−1peak indicated inFig. 1bis obscured by the surface plot colour scaling and is more easily seen inFig. 1b. Figure 3: Surface plots of Δabs versus protein crystal orientation angle and frequency. ( a ) Hydrated CEWL crystal CATM measurements. ( b ) Hydrated CEWL crystal normal mode calculations. The measurements show the same periodicity as predicted by the calculations. The dashed lines indicate frequencies where measured periodic peaks have frequencies similar to periodic peaks in the calculations. The calculated 47 cm −1 peak indicated in Fig. 1b is obscured by the surface plot colour scaling and is more easily seen in Fig. 1b . Full size image In Fig. 3b we replot the Δabs calculations shown in Fig. 1b as a surface plot, allowing direct comparison with the measurement. The colour scaling in Fig. 3b obscures the 23 and 47 cm −1 peaks seen in Fig. 1b . The measured angular dependence in Fig. 3a agrees with the calculated angular dependence in Fig. 3b . Comparison with the calculated spectra suggests that the measured orientation-dependent Δabs peaks of the hydrated crystal at 12, 20, 45, 69 and 78 cm −1 may correspond to the calculated modes at 8, 23, 47, 67 and 80 cm −1 , respectively. While computational methods are becoming more precise, it appears somewhat optimistic to expect strong frequency-dependent agreement with spectroscopy using current methods. However, by performing calculations and measurements in concert as a function of ligand binding and mutation, one might identify modes through consistent changes in frequency and/or amplitude. That is, in the case of CEWL, a specific set of modes associated with hinge motion will no longer be accessible with the inhibitor present. These modes would then be identified by their presence in the free protein and absence in the inhibitor-bound protein sample. CEWL crystal measurements were previously attempted using THz time domain spectroscopy (THz TDS) [27] . Those measurements were performed in the far field as a function of hydration, and no resonances associated with the protein were observed. Far-field diffraction likely obscured the strong absorbances that we report here. The sharp orientation-dependent resonances may originate from either intramolecular motions or crystal lattice vibrations, phonons. Typical molecular crystals (such as sucrose) with basis group molecular weights of ~100 Da have lattice phonons in the 10–100 cm −1 range [29] , [30] , [31] . The lattice phonon frequency will scale inversely with the square root of the mass of the lattice basis, suggesting the lattice phonons for the 14-kDa molecular weight CEWL basis crystals are over an order of magnitude smaller, with frequencies less than 10 cm −1 . Indeed, recent protein crystal phonon dispersion calculations for RNase using an all-atom treatment found that the highest frequency optical mode with lattice phonon dispersion was at 10 cm −1 (ref. 32 ). All higher frequency optical modes were independent of the lattice indicating intramolecular vibrations. RNase is a 124 residue protein similar in size to the 129 residue lysozyme. The RNase calculation did not include anharmonicity and damping, which would further red shift the lattice phonons far below the resonances reported here. Previous Raman measurements also support that the modes observed with CATM are intramolecular vibrations [33] , [34] . Of particular note is the previous observation of a hydration-independent CEWL crystal Raman shoulder at 45 cm −1 , which may correspond to the sharp peak observed here [34] . It is interesting to consider previous Raman and far-infrared measurements, which provide evidence that the features observed in the CATM results arise from intramolecular motions. Early Raman measurements of lysozyme crystals found broad shoulders on the main Rayleigh peak at 25, 75, 115 and 160 cm −1 (ref. 33 ). As the 25 cm −1 line was absent in solution-phase measurements, the authors concluded that this mode is a phonon; however, they also suggested the 25 cm −1 mode could be an internal mode of lysozyme that was strongly damped in solution. The 75 cm −1 shoulder was also found in solution-phase measurements and was therefore associated with an intramolecular vibration. More recent measurements on wet and dry lysozyme crystals found distinct, although broad peaks, at 17±7, 45±48, 85±66, 112±35 and 183±270 cm −1 (ref. 34 ). These resonances were nearly independent of scattering geometry. The spectra were not measured as a function of excitation polarization, which would be complimentary to the CATM measurements. The lack of dependence on scattering geometry led the authors to conclude that the observed modes must be intramolecular and not crystal phonons. Of particular interest is the 45 cm −1 mode, which had little dependence on hydration. For these low symmetry molecules, vibrational modes may be both optically and Raman active, suggesting that this Raman mode may be identical to the 45 cm −1 mode found using CATM for both wet and dry crystals. In addition to the Raman measurements, there has previously been a report of a possible intramolecular absorbance at 19 cm −1 for CEWL powder hydrated to 0.1 g H 2 O per g protein that diminished as the sample was hydrated [35] . In that work, Fourier transform interferometry measurements used a synchrotron source with a spectral range of 15–45 cm −1 . It is possible that this is the same 19 cm −1 mode that CATM detects in the dry protein crystals. The strong CATM feature at 45 cm −1 was not observed in the synchrotron measurements; however, this may be because the frequency is at the edge of the measurement range for those earlier measurements. The CATM linewidths are somewhat surprisingly narrow (~5 cm −1 ), compared with the measured Raman linewidths. Often it is assumed that the large-scale internal vibrational motions for proteins will be overdamped. However, there have been few quantitative studies of the actual damping. For partially hydrated powders, a set of normal mode calculations of the neutron-scattering intensity using Langevin damping as a function of frequency for bovine pancreatic trypsin inhibitor had best agreement with experimental results for overdamping of modes below 25 cm −1 (ref. 36 ). Only one publication has presented a calculation of the mode damping as a function of mode for a protein crystal [37] . The calculation found for modes greater than 17 cm −1 are in fact underdamped. While our measurements on lysozyme crystals are consistent with that result, the calculation still predicted somewhat larger linewidths than the CATM technique measures. It is possible that the narrow linewidths observed with CATM result from employing Δabs, which will amplify and sharpen features as is the case for time-resolved optical pump-infrared probe vibrational measurements [38] . We note that a previous far-infrared pump/probe measurement suggested that extremely long-lived low-frequency excitations are present for bacteriorhodopsin [39] . In conclusion, optical measurements at terahertz frequencies find that underdamped large-scale correlated motions exist for proteins for frequencies greater than 10 cm −1 , lower than the cutoff predicted by normal mode calculations [36] and principal component calculations [37] . The CATM method introduced here enables the identification of protein-correlated structural motions. Implementation of this method is the first step towards determining the functional relevance of these motions. For example, specific mutations and binding can be used to restrict a particular mode identified by CATM. Subsequent measurements on reaction rates can then reveal if the mode is functionally relevant. Such a combined approach can potentially reveal structural dynamics mechanisms of ligand binding and allosteric control. Spectroscopic methods THz TDS has become a standard spectroscopic method in this frequency range [40] , [41] . Terahertz pulses are generated and detected coherently giving a time-dependent field profile E ( t ). The Fourier transform then gives the frequency content with amplitude and phase E (ω) e iϕ (ω) . The wavelength range is λ =50 μm–1 mm. Given that typical protein crystals have dimensions ~100 μm, far-field optical measurements are challenging owing to the diffraction limited spot size for this frequency range is 500 μm. To overcome this limitation, we use a THz TDS near-field scanning microscope method based on that by Planken [42] . This approach uses standard photoconductive THz generation and electro-optic detection [43] , [44] ; however, for THz near-field scanning microscope, the sample is placed directly on top of a horizontal ZnTe electro-optic detection crystal. A near-infrared probe is used to detect the THz light. This near-infrared beam is incident from the back of the electro-optic crystal and its spot size determines the image resolution. The spatial resolution of our system is 10–30 μm. The THz system is enclosed and purged with dry nitrogen to remove artifacts from gas-phase water. All measurements are performed at room temperature. To ensure that the protein crystal remains in a hydrated atmosphere, the ZnTe crystal forms part of a humidity-controlled chamber for the sample. The hydration in the chamber is controlled by a flow from a Licor Dewpoint generator set to 100% relative humidity. If a protein crystal sample is placed directly on the ZnTe electro-optic crystal, the radiation detected is both that transmitted through the sample and that diffracted by sample edges. The contamination from diffraction is sufficiently large that absorption peaks can be entirely obscured. Knab et al. [45] demonstrated that by using small apertures one can attain the same spectroscopic quality from microscopic samples in the near field as can be achieved in the far field for macroscopic samples. We implement this method by mounting the protein crystals over a 300-μm diameter aperture in a thin aluminium plate (~150 μm thick). Different orientations are measured by rotating this sample plate. A THz image is acquired by scanning the ZnTe-sample stage and measuring a THz waveform for each pixel. For each orientation angle, a THz image is taken of the aperture to determine the centre pixel positions, which will change slightly owing to the manual rotation of the sample plate. The Δabs spectra are determined from the centre pixels for each orientation. A typical transmission measurement consists of measuring the transmitted field through a reference and the sample giving the field transmittance: where f ( ω ) is the loss from Fresnel reflection, α (ω) is the absorption coefficient, c is the speed of light, n ( ω ) is the refractive index and d is the sample thickness. Challenges in determining the frequency-dependent absorbance in the THz region include proper referencing and removal of multiple reflection interference effects, often referred to as the Fabry–Perot etalon. We address both the referencing and etalon concerns by self referencing. As we are interested in the change in absorbance with orientation, we use a single orientation of the crystal as our reference and calculate a difference absorbance using the following: where | E t ( ω,θ )| (| E i ( ω,θ )|) is the magnitude of the transmitted (incident) electric field, α ( ω , θ ) is the sample’s absorption coefficient at frequency ω , orientation angle θ , and d is the sample thickness. F ( ω ) is the frequency-dependent transmission due to Fresnel loss at interfaces, subwavelength aperture effects and etalon. This factor should be orientation independent. By using the centre pixels of the aperture at a given orientation, we ensure that the thickness of the sample is always the same, even for a faceted crystal; thus, the removal of etalon should be valid as long as there is no strong birefringence. As we are measuring the anisotropic response of the crystal, it is important that the linear polarization of the THz light is preserved for the measurement. We find that the polarization remains linear and the spectral content does not change for the central pixels of the aperture, and only at the edges of the aperture does one observe the field lines bending to the normal of the circular metal aperture and deviation from the frequency content at the centre pixels. In the case of the dehydrated crystal, the magnitude of the transmission spectra was scaled by a constant frequency-independent factor to account for possible inhomogeneities in the ZnTe crystal or system drift between rotations. It was subsequently determined that this scaling was not necessary, and was not performed for the hydrated crystal data. This overall measurement technique with self referencing, we refer to as CATM. CATM characterization Spectroscopic testing of an anisotropic standard is done with sucrose crystals discussed in the Supplementary Methods and with Supplementary Fig. 2 . The calibration measurements demonstrate that the technique has both excellent spectral reproducibility and is free from etalon contamination. Sample methods CEWL crystals are grown using the sitting drop method. The protein is supplied by Sigma-Aldrich and used at 60 mg ml −1 in 0.1 M NaAc pH 5.2 buffer without further purification. The precipitant is 10% NaCl in the same buffer. The sitting drop contained 10 μl of precipitant and 10 μl of protein solution with 500 μl of precipitant in the reservoir. Crystals grow over a period of a few days. Tetragonal crystals, space group P4 3 2 1 2, are mounted on the sample plate and then the plate is placed in the hydration chamber atop the ZnTe detection crystal. Measurements are performed on ‘dry’ crystals and ‘wet’ crystals. In the case of the ‘dry’ crystals, the crystal is simply placed over the aperture of the sample plate without any paraffin oil. The dry crystals maintain their initial facets; however, internal cracking is apparent. For ‘wet’ crystals, a thin polypropylene sheet is stretched and glued to the back of the sample plate. The crystal is then mounted over the aperture of the plate and immediately covered with paraffin oil. The thickness of the paraffin coating is <10 μm. The measured transmission of paraffin oil is flat over 0.2–3.0 THz with and estimated absorption coefficient ~10 cm −1 . The THz is incident on the (110) face; thus, the terahertz polarization vector lies in the plane perpendicular to [110]. Modelling methods Optical measurements have the potential to decrease the complexity of the dense VDOS by optical selection rules. Optically active excitations require a dipole change with the excitation. The result is that, unlike inelastic neutron measurements, which measure the complete VDOS, the optical response reflects the mode-dependent dipole coupling with possibly some modes having no coupling at all, resulting in more structure in the spectrum and possible mode identification. Typical optical measurements are limited to macroscopic samples (solutions, powders and films) of randomly aligned molecules and what is measured is the absorption averaged over all orientations, which is given by: where , ω i and γ i are the dipole derivative, mode frequency and linewidth associated with mode i , respectively. abs isotropic is an additional glass-like background from librational motions of the solvent and peptide side chains. These local motions are not reproduced in the normal mode spectrum, shown in Fig. 1a . The utility of using crystal anisotropy to remove the glass-like contribution is clear from the general absorption equation for a single molecule: where is the unit vector in the direction of the polarization of the incident light. Unlike in equation (3) where the response is averaged over all orientations, the first term in equation (4) is dependent on the orientation of the molecule relative to the light polarization direction. The second term is the same as in equation (3) and is independent of the polarization direction, and will be removed when the absorption difference is calculated for two different orientations. For example, if the polarization is initially in the x direction for the coordinate system of the protein, and is then rotated in the x – y plane by angle θ , the change in the absorption as a function of orientation angle is independent of the isotropic contribution: Single-molecule measurements are not yet possible at terahertz frequencies. To measure this contrast with orientation, an assembly of ordered molecules needs to be measured. Here protein crystals provide this ordered assembly. In general, for crystals, the molecules are not absolutely and uniformly aligned, but instead for a single-unit cell there are typically several replica molecules translated and rotated corresponding to the crystal symmetry group. In addition, the crystal formation itself indicates there are crystal contact forces that may need to be accounted for in the calculation of the collective vibrations. Ideally, to calculate Δabs then one would calculate the spectrum for the crystal as was done for RNase [32] using normal mode analysis (NMA) or staphylococcal nuclease using principal component analysis [37] . Those calculations included all proteins and waters in the unit cell, and were the first attempts to include crystal contact forces. However, there is some evidence that crystal contact forces are weak [32] , [46] and as we are interested in the intramolecular motions rather than the lattice phonons, we assume zero-crystal contact forces and calculate the net crystal response by summing the single-molecule response over the unit cell, accounting for the molecular rotations for the crystal symmetry group: where is a rotation matrix associated with the crystal symmetry. This simplification allows us to first introduce the overall methodology of the spectrum calculation, which can be improved by performing the principal component analysis for a multi-cell crystal at room temperature. We perform NMA to calculate the hydrated single-molecule VDOS and the dipole derivatives using version 32 of CHARMM [47] with all-atom parameter set 22 (ref. 48 ). The X-ray structure file 1bwh.pdb is used as the starting structure. The 92 crystal waters are included using TIP3 (TIP3p) explicit solvent. The structure is minimized at zero temperature using several iterations of 2,000 steps of adopted basis Newton Raphson method and then 20,000 steps of Newton Raphson and another 20,000 steps of steepest descent until the energy gradient was 10 −6 kcal Å −1 . The energy-minimized structure is then used for NMA using the VIBRAN command, which determines the eigenfrequencies, eigenvectors and net dipole derivative for each vibrational mode. The dipole derivative assumes fixed partial charges. We calculate the expected anisotropic response using the first term in equation (6) for the polarization rotated perpendicular to [110], the rotation matrices for space group P4 3 2 1 2 and a single linewidth γ =4 cm −1 . We reference the spectra to the polarization direction, along the [−110] direction. How to cite this article: Acbas, G. et al. Optical measurements of long-range protein vibrations. Nat. Commun. 5:3076 doi: 10.1038/ncomms4076 (2014).